Cyclin D1 induction of Dicer governs microRNA processing and expression in breast cancer C yclin D1 encodes the regulatory subunit of a holoenzyme that phosphorylates the pRB protein and promotes G 1 /S cell-cycle progression and oncogenesis. Dicer is a central regulator of miRNA maturation, encoding an enzyme that cleaves double-stranded RNA or stem–loop–stem RNA into 20–25 nucleotide long small RNA, governing sequence-specific gene silencing and heterochromatin methylation. The mechanism by which the cell cycle directly controls the non-coding genome is poorly understood. Here we show that cyclin D1 −/− cells are defective in pre-miRNA processing which is restored by cyclin D1a rescue. Cyclin D1 induces Dicer expression in vitro and in vivo . Dicer is transcriptionally targeted by cyclin D1, via a cdk-independent mechanism. Cyclin D1 and Dicer expression significantly correlates in luminal A and basal-like subtypes of human breast cancer. Cyclin D1 and Dicer maintain heterochromatic histone modification (Tri-m-H3K9). Cyclin D1-mediated cellular proliferation and migration is Dicer-dependent. We conclude that cyclin D1 induction of Dicer coordinates microRNA biogenesis. MicroRNAs (miRNAs), a class of non-coding small RNA, are initially transcribed to primary-miRNA (pri-miRNA), which are then cleaved by the endonuclease Drosha and its partner DGCR8 to generate hairpin-folded pre-miRNAs of 60–70 nucleotides in length [1] . Following transport to the cytoplasm by Exportin-5, pre-miRNAs are processed by Dicer with its partner TRBP ((HIV-1 transactivating response (TAR) RNA-binding protein) to generate the 20–22 nucleotide mature miRNAs [1] , [2] , [3] , [4] . Mature miRNAs then associate with Argonaute (Ago) proteins to regulate target mRNA expression through the RNA-induced silencing complex. miRNAs regulate gene expression through base-pair binding to the complementary sequence in the 3′ untranslated region (3′ UTR) of mRNA. miRNAs contribute to the timing of development, apoptosis, cell-cycle progression, cellular proliferation, stem cell self-renewal, cancer initiation and metastasis [5] , [6] , [7] , [8] . The expression of miRNA is regulated during cell-cycle transition and cellular contact in part via active degradation [9] . Aberrant expression of miRNAs or mutations of miRNA genes have been described in many types of tumours, including mammary tumours [10] . The RNase III endoribonuclease Dicer cleaves long double-stranded RNA or stem-loop-stem structured pre-miRNA to form mature miRNAs. RNAi-mediated knockdown of Dicer in human cells led to defects in both miRNA production and shRNA-mediated RNAi [11] , [12] . Drosophila Dicer mutant germline stem cells are delayed in the G 1 –S transition and are defective in cell-cycle control [13] . Dicer expression is induced during keratinocyte differentiation via MITF (micropthalmia-associated transcription factor (TF)) [14] . Tissue-specific knockout of Dicer demonstrated a role in murine cellular growth, differentiation, development and stem cell maintenance [15] . Initially cloned as a breakpoint rearrangement in parathyroid adenoma, the cyclin D1 gene encodes the regulatory subunit of the holoenzyme that phosphorylates and inactivates both the pRb tumour suppressor and the key inducer of mitochondrial biogenesis NRF-1 (refs 16 , 17 ). In addition, a DNA bound form of cyclin D1 regulates gene expression [18] , [19] , [20] . Cyclin D1 expression is induced during mammary gland and retinal differentiation, and deletion of the murine cyclin D1 gene resulted in failed terminal alveolar breast bud development and retinal degeneration. Diverse biological functions regulated by cyclin D1 include the induction of cellular proliferation, angiogenesis, cellular migration, DNA damage repair, mitochondrial biogenesis, stem cell maintenance and miRNA expression [3] , [21] . Cyclin D1 was shown to regulate the miR-17/20 locus and found to bind the miR-17/20 regulatory region (3). In this study, in order to determine further the mechanism by which cyclin D1 regulates non-coding RNA, we conducted studies of miRNA processing. We established cyclin D1 −/− mouse embryonic fibroblasts (MEFs) cells and cyclin D1 knockdown (KD) MCF-7 human breast cancer cells. miRNA analysis indicated an induction of mature miRNA expression in cyclin D1 overexpressing cells. Analysis of the miRNA-processing regulators demonstrated the selective induction of Dicer expression by cyclin D1. In cyclin D1 −/− cells, the reduction of Dicer abundance was accompanied by the impairment of pre-miRNA to mature miRNA processing, which was restored with cyclin D1 rescue. Transient transgenic expression of cyclin D1 in the mouse mammary gland, or sustained transgenic expression of cyclin D1 -induced mouse mammary gland tumours, recapitulated the induction of Dicer expression. Cyclin D1 and Dicer expression were correlated in luminal A and basal-like human breast cancer. Cyclin D1 regulation of cellular proliferation and migration was dependent upon Dicer. By demonstrating cyclin D1-induced Dicer abundance and function in tissue culture and in vivo , we provide evidence for crosstalk between the cell-cycle and non-coding miRNA biogenesis. Cyclin D1 induces Dicer expression In our prior studies demonstrating cyclin D1 induction of the miR-17/20 locus [22] , we observed altered abundance of miR-17/20 precursor versus mature miRNA abundance in breast cancer cell lines associated with altered expression of cyclin D1. In addition, miRNA analysis in cyclin D1 −/− and cyclin D1 restored MEF cells demonstrated the induction of miRNA abundance by cyclin D1a [22] . We examined the possibility that cyclin D1a may regulate miRNA biogenesis. Key regulators for each step of miRNA processing were analysed in wild-type (WT) and cyclin D1 siRNA-treated MCF-7 human breast cancer cells ( Fig. 1a ). Drosha and DGCR8, two essential components of the pri-miRNA processing complex [23] , Ago2, a key component of the siRNA/miRNA-induced gene silence complex, and Exportin 5, which mediates nuclear export of pre-miRNAs to cytoplasm [2] , did not show regulation by cyclin D1 ( Fig. 1a,b ). Dicer was downregulated in cyclin D1 -deficient MCF-7 cells ( Fig. 1a,c ). In order to determine whether cyclin D1 induces Dicer in vivo, we examined the Dicer mRNA and protein level in the mammary gland from tetracycline-inducible MMTV- cyclin D1 transgenic mouse. The transient induction of the mammary epithelial cell-targeted cyclin D1 transgene expression for 1 week was sufficient for the induction of Dicer expression (~4-fold, N =3 separate mice) ( Fig. 1d,e ). MMTV- cyclin D1 -induced mouse mammary gland tumours also showed increased Dicer mRNA abundance ( Fig. 1f ). Dicer promoter luciferase reporter assays combined with knockdown of endogenous cyclin D1 in MCF-7 cells or overexpression of cyclin D1 in 293T cells demonstrated activation of the Dicer promoter by cyclin D1a ( Fig. 1g,h ). Moreover, this induction of Dicer was cyclin D1 kinase-binding domain independent as expression of the cyclin D1 KE mutant, which lacks the ability to activate cyclin D1-dependent kinase activity, induced Dicer promoter luciferase activity to a similar level as WT cyclin D1a ( Fig. 1h ). As a negative control, the basic luciferase reporter vector backbone lacking the Dicer promoter did not show significant change in the luciferase activity upon co-transfection of expression vectors for either cyclin D1a or cyclin D1 KE ( Fig. 1h ). 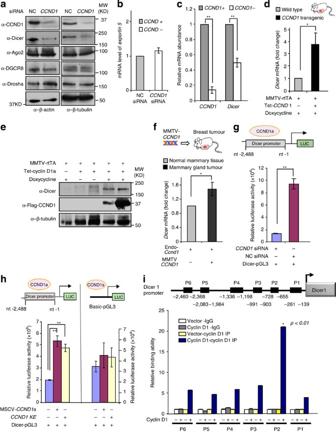Figure 1: Endogenous cyclin D1 maintains Dicer expression. (a) Western blot showing decreased Dicer abundance in the cyclin D1 siRNA-treated MCF-7 cells. Antibodies are directed to the miRNA biogenesis proteins Dicer, Ago2, DGCR8 and Drosha. (b) Real-time PCR analysis ofExportin 5mRNA in MCF-7 cells treated with cyclin D1 siRNA or control siRNA. Values are equal to mean ±s.e.m. (N=3). No significant difference between two samples by the standard two-tailed Student’st-test. (c) Real-time PCR demonstrating decreased cyclin D1 and Dicer mRNA level in the cyclin D1 siRNA-treated MCF-7 cells. Values are equal to mean ±s.e.m. ofN=3 separate experiments. **P=0.0013 (cyclin D1) and 0.0026 (Dicer). Statistical significance was determined by the standard two-tailed Student’st-test. (d) Dicer mRNA abundance induced in the mammary gland of tet-inducable MMTV-cyclin D1a transgenic mice treated with doxycycline for 1 week. Data are mean ±s.e.m. forN=3 separate transgenic mice *P=0.0334 (standard two-tailed Student’st-test). (e) Dicer protein level in mammary gland tumours of tet-inducible MMTV-cyclin D1a transgenic mice treated with doxycycline. (f) Dicer mRNA in mammary gland tumours of MMTV-cyclin D1a transgenic mice with comparison to age matched mammary gland. Data are mean±s.e.m. for three separate transgenic tumours and three normal mammary glands. *P=0.0308 (standard two-tailed Student’st-test). (g) Luciferase activity for the Dicer promoter in MCF-7 cells. Cells were treated with control and cyclin D1 siRNA as indicated. Data are mean ±s.e.m. for triplicates inN=3 separate transfections normalized to β-galactosidase reporter activity. **P<0.001. (h) Relative luciferase activity of the Dicer promoter and vector control in the presence of an expression vector for either cyclin D1 or a kinase-defective mutation (cyclin D1 KE). Data are shown as mean ±s.e.m. forN=3 separate transfections. **P=0.0083 (cyclin D1a) and 0.0033 (cyclin D1KE). Statistical significance was determined by the standard two-tailed Student’st-test. (i) Cyclin D1 ChIP analysis revealed the specific binding to a region (−728 to −655) of the Dicer promoter. Both IgG IP to cyclin D1-overexpressing cells and cyclin D1-Flag IP to control cells were performed as negative control. Figure 1: Endogenous cyclin D1 maintains Dicer expression. ( a ) Western blot showing decreased Dicer abundance in the cyclin D1 siRNA-treated MCF-7 cells. Antibodies are directed to the miRNA biogenesis proteins Dicer, Ago2, DGCR8 and Drosha. ( b ) Real-time PCR analysis of Exportin 5 mRNA in MCF-7 cells treated with cyclin D1 siRNA or control siRNA. Values are equal to mean ±s.e.m. ( N =3). No significant difference between two samples by the standard two-tailed Student’s t -test. ( c ) Real-time PCR demonstrating decreased cyclin D1 and Dicer mRNA level in the cyclin D1 siRNA-treated MCF-7 cells. Values are equal to mean ±s.e.m. of N =3 separate experiments. ** P =0.0013 (cyclin D1) and 0.0026 (Dicer). Statistical significance was determined by the standard two-tailed Student’s t -test. ( d ) Dicer mRNA abundance induced in the mammary gland of tet-inducable MMTV-cyclin D1a transgenic mice treated with doxycycline for 1 week. Data are mean ±s.e.m. for N =3 separate transgenic mice * P =0.0334 (standard two-tailed Student’s t -test). ( e ) Dicer protein level in mammary gland tumours of tet-inducible MMTV-cyclin D1a transgenic mice treated with doxycycline. ( f ) Dicer mRNA in mammary gland tumours of MMTV-cyclin D1a transgenic mice with comparison to age matched mammary gland. Data are mean±s.e.m. for three separate transgenic tumours and three normal mammary glands. * P =0.0308 (standard two-tailed Student’s t -test). ( g ) Luciferase activity for the Dicer promoter in MCF-7 cells. Cells were treated with control and cyclin D1 siRNA as indicated. Data are mean ±s.e.m. for triplicates in N =3 separate transfections normalized to β-galactosidase reporter activity. ** P <0.001. ( h ) Relative luciferase activity of the Dicer promoter and vector control in the presence of an expression vector for either cyclin D1 or a kinase-defective mutation (cyclin D1 KE). Data are shown as mean ±s.e.m. for N =3 separate transfections. ** P =0.0083 (cyclin D1a) and 0.0033 (cyclin D1KE). Statistical significance was determined by the standard two-tailed Student’s t -test. ( i ) Cyclin D1 ChIP analysis revealed the specific binding to a region (−728 to −655) of the Dicer promoter. Both IgG IP to cyclin D1-overexpressing cells and cyclin D1-Flag IP to control cells were performed as negative control. Full size image Recent studies had demonstrated a DNA bound form of cyclin D1 which participated in gene regulation [19] . In order to identify candidate cyclin D1-associated regions of the Dicer gene, we reinterrogated ChIP-Seq analysis conducted of cyclin D1 −/− MEFs transduced with a retroviral vector encoding FLAG-tagged cyclin D1 (ref. 19 ). We first examined the cyclin D1-associated chromatin of the Top2a gene, which had been identified in chromosomal immuno-precipitation (ChIP) as a target of cyclin D1-induced gene expression [19] ( Supplementary Fig. S1A ). The Dicer regulatory region analysis demonstrated a similar enrichment of cyclin D1-binding in chromatin by ChIP-Seq ( supplementary Fig. S1B ). We therefore examined at a high level of resolution the maximal region of enrichment for cyclin D1 chromatin association within the Dicer regulatory region. The region of −728 to −655 demonstrated a 20-fold enrichment of cyclin D1 association in the context of chromatin compared with other regions ( Fig. 1i ). The cyclin D1-associated region of the Dicer promoter includes several cis elements for TF binding. Many of these TF sites were also identified in the minimal cyclin D1 binding region of the miR-17/20 promoter ( Supplementary Fig. S1C ). In order to determine the importance of the P2 region to Dicer promoter activity in MCF-7 cells, comparison was made of Dicer promoter activity upon deletion of the P2 region. The relative activity of the Dicer promoter was reduced 2-fold upon deletion of the P2 region ( Supplementary Fig. S2 ). In order to define further the role of the cyclin D1-associated kinase activity and the domains of cyclin D1 required for the induction of Dicer abundance, cyclin D1 −/− MEFs were transduced with cyclin D1 WT and a mutant encoding a deletion of the C-terminus (N1) ( Supplementary Fig. S3 ). Western blot demonstrated an increase in Dicer abundance in the WT cells and a 60% reduction in the induction of Dicer by the N1 mutant of cyclin D1 ( Supplementary Fig. S3B ). Western blot with an antibody directed to the N-terminal FLAG tag of the cyclin D1 expression vectors demonstrated that the N1 mutant was expressed ~2-fold better than the cyclin D1 WT ( Supplementary Fig. S3B ). The N1 mutant was capable of enhanced binding to Cdk4 compared with WT cyclin D1 ( Supplementary Fig. S3C ). Together these studies suggest that the Cdk-binding domain of cyclin D1 can be dissociated from its ability to induce the expression of Dicer. Cyclin D1 restores pre-miRNA processing Dicer has a key role in the conversion of pre-miRNA to mature miRNA. Northern blot analysis was therefore conducted to examine representative examples of pre-miRNA and mature miRNA in WT and Dicer −/− cells, as well as in WT and cyclin D1 −/− cells. Comparison of miRNA processing was made between Dicer −/− , cyclin D1 −/− and cyclin D1 restored cells. The HCT116 Dicer −/− cells encode a targeted disruption of Dicer exon5 (ref. 24 ). In Dicer −/− cells, conversion of pre-miRNA (pre-miR-16, pre-let-7a, pre-miR-17 and pre-miR-20a) to mature miRNA (miR-16, let-7, miR-17 and miR-20a) was compromised ( Fig. 2a ). Similarly, pre-miR-16 processing was compromised in cyclin D1 −/− cells ( Fig. 2b lane 2 versus 1), which was rescued by either cyclin D1 restoration or Dicer re-expression ( Fig. 2b lanes 3 and 4 versus 2). The defect in processing of other representative miRNAs, including let-7, miR-17 and miR-20a, was observed in Dicer −/− ( Fig. 2a ) and cyclin D1 −/− cells ( Fig. 2c–e ). In order to further demonstrate the induction of miRNA expression and processing by cyclin D1a via Dicer, a vector expressing the human Dicer gene was used ( Supplementary Fig. S4A ). We conducted Dicer and cyclin D1 rescue of cyclin D1 −/− MEFs. Dicer or cyclin D1 transduction of cyclin D1 −/− cells was sufficient to restore expression and processing of representative miRNAs ( Fig. 2b–e ). 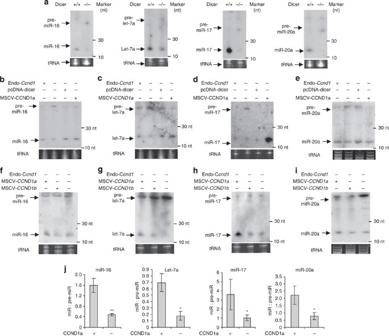Figure 2: Dicer or cyclin D1 expression rescues the processing of pre-miRNA to mature miRNA incyclin D1−/−cells. (a) Northern blot analysis of representative miRNAs (miR-16, let-7, miR-17 and miR-20a) in WT andDicer−/−HCT116 cells. (b–e) Northern blot analysis of pre-miR-16, pre-let-7a, pre-miR-17 and 20a to mature miRNA processing incyclin D1+/+,cyclin D1−/−andcyclin D1−/−MEFs reintroduced with Dicer orcyclin D1a. (f–i) Northern blot detection of pre-let-7a, pre-miR-16, 17 and 20a and mature let-7a, miR-16, 17 and 20a in cyclin D1a (lane 1) and cyclin D1b (lane 2) rescuedcyclin D1−/−MEFs (lane 3). (j) Quantitative analysis of pre-let-7a, pre-miR-16, 17 and 20a to mature let-7a, miR-16, 17 and 20a processing incyclin D1−/−andcyclin D1+/+MEFs. Values are equal to mean±s.e.m. (n=3). **P=0.0075 (miR-16), *P=0.0143 (let-7a), 0.05012 (miR-17) and 0.0472 (miR-20a). Statistical significance was determined by the standard two-tailed Student’st-test. tRNA serves as a loading control for northern blot. Figure 2: Dicer or cyclin D1 expression rescues the processing of pre-miRNA to mature miRNA in cyclin D1 − / − cells. ( a ) Northern blot analysis of representative miRNAs (miR-16, let-7, miR-17 and miR-20a) in WT and Dicer −/− HCT116 cells. ( b – e ) Northern blot analysis of pre-miR-16, pre-let-7a, pre-miR-17 and 20a to mature miRNA processing in cyclin D1 +/+ , cyclin D1 −/− and cyclin D1 −/− MEFs reintroduced with Dicer or cyclin D1a . ( f – i ) Northern blot detection of pre-let-7a, pre-miR-16, 17 and 20a and mature let-7a, miR-16, 17 and 20a in cyclin D1a (lane 1) and cyclin D1b (lane 2) rescued cyclin D1 −/− MEFs (lane 3). ( j ) Quantitative analysis of pre-let-7a, pre-miR-16, 17 and 20a to mature let-7a, miR-16, 17 and 20a processing in cyclin D1 −/− and cyclin D1 +/+ MEFs. Values are equal to mean±s.e.m. ( n =3). ** P =0.0075 (miR-16), * P =0.0143 (let-7a), 0.05012 (miR-17) and 0.0472 (miR-20a). Statistical significance was determined by the standard two-tailed Student’s t -test. tRNA serves as a loading control for northern blot. Full size image The rescue of Cyclin D1 −/− cells via transduction with a cyclin D1 expressing retrovirus ( Supplementary Fig. S4B ) increased the conversion of pre-miRNA to mature miRNA ( Fig. 2f–i and Supplementary Fig. S5 ). Transduction of cyclin D1 −/− cells with a retroviral expression vector encoding cyclin D1a restored processing of pre-miR-16 to mature miR-16 ( Fig. 2b lane 4 versus lane 2 and Fig. 2f lane 1 versus lane 3). Similarly, increased processing of pre-let-7a, pre-miR-17 and pre-miR-20a was observed in the cyclin D1a rescued cells ( Fig. 2c–e lane 4 versus lane 2 and Fig. 2g–i lane 1 versus lane 3). Consistent with the reduction in Dicer abundance, the relative conversion of pre-let-7a, pre-miR-16, 17 and 20a to mature let-7a, miR-16, 17 and 20a was reduced in cyclin D1 −/− cells. The ratio of mature form to precursor form of the detected miRNAs was 3–5-fold higher in cyclin D1 +/+ cells than in cyclin D1 −/− cells ( Fig. 2j ). Cyclin D1 and Dicer maintain histone tri-methylation In Schizosaccharomyces pombe, Dicer regulates small RNA from pericentric repeats that initiate histone H3 lysine (H3K9) methylation and heterochromatin formation at these domains. Dicer 1-deficient mouse embryonic stem cells have decreased H3K9 trimethylation and decreased DNA methylation [25] , [26] . In order to examine further the functional significance of cyclin D1-dependent induction of Dicer, we examined the hetero-chromatic histone modification previously attributed to Dicer [26] . Consistent with prior findings in Dicer −/− ES cells, HCT116 Dicer −/− cells demonstrated reduced tri-m-H3K9 immunofluorescence ( Fig. 3a ). Cyclin D1 siRNA treatment of HCT116 resulted in a similar reduction in tri-m-H3K9 immunofluorescence as observed with Dicer1 genetic deletion ( Fig. 3a ). Cyclin D1 siRNA treatment of Dicer −/− HCT116 cells resulted in a further reduction in tri-m-H3K9 immunofluorescence ( Fig. 3a ). Consistent with the reduction in Dicer abundance in cyclin D1 −/− MEFs, the tri-m-H3K9 immunofluorescence was reduced in cyclin D1 −/− MEFs ( Fig. 3b ). Similarly, reduced tri-m-H3K9 expression was observed in cyclin D1 knockdown MCF-7 cells ( Fig. 3c ), where Dicer expression was reduced ( Fig. 1a ). The Dicer loss in Dicer −/− HCT116 cells and cyclin D1 loss in cyclin D1 −/− MEFs were demonstrated by western blot analyses ( Fig. 3d,e ). 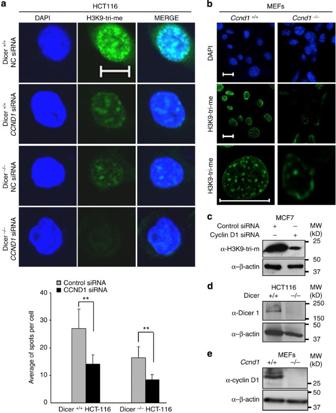Figure 3: Dicer and cyclin D1 govern heterochromatic H3K9 trimethylation. (a) HCT116 cells were stained with an antibody specific for trimethyl-H3K9 and DAP1 strained for nuclei. H3K9 trimethylation was assessed inDicer+/+versusDicer−/−HCT116 cells treated with cyclin D1 siRNA or control. Quantitative analysis of trimethyl-H3K9 induction by Dicer and cyclin D1 was indicated. Scale bars, 10 μm. mean ±s.e.m. representing H3K9-Tri-me staining spots in 10 randomly selected cells. **P=0.0015 for WT HCT116, and 0.0078 for Dicer−/−HCT116. The experiments were repeated independently for three times. Statistical significance was determined by the standard two-tailed Student’st-test. (b) H3K9 trimethylation was assessed incyclin D1+/+versuscyclin D1−/−MEFs. Scale bars, 10 μm. (c) Western blot for trimethyl-H3K9 in control and cyclin D1 siRNA treated MCF-7 cells. (d) Western blot for Dicer in WT andDicer−/−HCT116 cells. (e) Western blot for cyclin D1 in WT andcyclin D1−/−MEFs. ß-actin served as a loading control in all western blot analysis. Figure 3: Dicer and cyclin D1 govern heterochromatic H3K9 trimethylation. ( a ) HCT116 cells were stained with an antibody specific for trimethyl-H3K9 and DAP1 strained for nuclei. H3K9 trimethylation was assessed in Dicer +/+ versus Dicer −/− HCT116 cells treated with cyclin D1 siRNA or control. Quantitative analysis of trimethyl-H3K9 induction by Dicer and cyclin D1 was indicated. Scale bars, 10 μm. mean ±s.e.m. representing H3K9-Tri-me staining spots in 10 randomly selected cells. ** P =0.0015 for WT HCT116, and 0.0078 for Dicer −/− HCT116. The experiments were repeated independently for three times. Statistical significance was determined by the standard two-tailed Student’s t -test. ( b ) H3K9 trimethylation was assessed in cyclin D1 +/+ versus cyclin D1 − / − MEFs. Scale bars, 10 μm. ( c ) Western blot for trimethyl-H3K9 in control and cyclin D1 siRNA treated MCF-7 cells. ( d ) Western blot for Dicer in WT and Dicer −/− HCT116 cells. ( e ) Western blot for cyclin D1 in WT and cyclin D1 −/− MEFs. ß-actin served as a loading control in all western blot analysis. Full size image Cyclin D1 mediates proliferation and migration via Dicer Cyclin D1 enhances cellular proliferation and cyclin D1 siRNA reduced HCT116 cellular proliferation assessed using the MTT (3-(4,5-dimethylthiazol-2-yl)-2,5-diphenyltetrazolium) assay ( Fig. 4a ). Cyclin D1 siRNA had no effect on cellular proliferation in Dicer −/− HCT116 cells ( Fig. 4a ), suggesting a requirement for Dicer in cyclin D1-induced cellular proliferation. 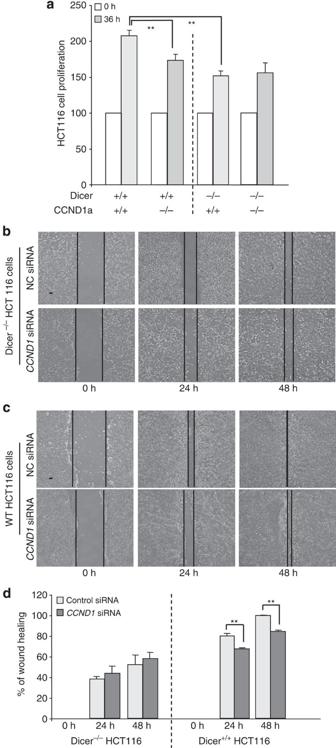Figure 4: Dicer-dependent cyclin D1-induced cellular proliferation and migration. (a) Cellular proliferation was assessed using MTT assays on HCT116Dicer+/+and HCT116Dicer−/−cells upon treatment with cyclin D1a siRNA or control siRNA as indicated. (b,c) Cellular migration assessed using wounding healing assays onDicer−/−(b) orDicer+/+(c) HCT116 cells upon treatment with cyclin D1 siRNA or control siRNA as indicated. Scale bars, 10 μm. (d) Quantitative analysis of the cellular migration assayed inbandc.a, Data are mean ±s.e.m. representing three separate experiments with triplicate for each (N=9). **P<0.001.d, Data are mean ±s.e.m. forN=3 separate experiments. **P=0.0032 for 24h, P<0.001 for 48h. Figure 4: Dicer-dependent cyclin D1-induced cellular proliferation and migration. ( a ) Cellular proliferation was assessed using MTT assays on HCT116 Dicer +/+ and HCT116 Dicer −/− cells upon treatment with cyclin D1a siRNA or control siRNA as indicated. ( b , c ) Cellular migration assessed using wounding healing assays on Dicer −/− ( b ) or Dicer +/+ ( c ) HCT116 cells upon treatment with cyclin D1 siRNA or control siRNA as indicated. Scale bars, 10 μm. ( d ) Quantitative analysis of the cellular migration assayed in b and c . a , Data are mean ±s.e.m. representing three separate experiments with triplicate for each ( N =9). ** P <0.001. d , Data are mean ±s.e.m. for N =3 separate experiments. ** P =0.0032 for 24h, P<0.001 for 48h. Full size image Dicer has cell-type-specific effects on migration as Dicer knockdown enhanced invasiveness of LKR13 cells [27] , Dicer had a dose-dependent effect in enhancing or inhibiting migration of MDA-MB-231 cells, and Dicer enhanced migration of T cells [28] . Cyclin D1 promotes cellular migration in a variety of cell types [29] , [30] . We examined the role of Dicer and cyclin D1 in HCT116 cell migration. Cyclin D1 knockdown reduced the rate of wound closure in HCT116 cells but had no effect on Dicer −/− HCT116 cells ( Fig. 4b–d ). In addition, Dicer −/− HCT116 cells demonstrated a reduced rate of wound closure compared with WT HCT116 cells ( Fig. 4b–d ). Thus cyclin D1-mediated cellular migration occurs through a mechanism that appears to require Dicer. These findings are consistent with prior studies demonstrating a role for miRNA in cyclin D1-mediated cell migration [22] . Cyclin D1 correlates with Dicer expression in breast cancer In order to analyse the association between Dicer and cyclin D1 expression in the context of breast cancer, a breast cancer microarray data set compiled [31] from the public repositories Gene Expression Omnibus ( http://www.ncbi.nlm.nih.gov/geo/ ) and Array Express ( http://www.ebi.ac.uk/arrayexpress/ ) was used to evaluate expression levels of Dicer and cyclin D1 in the context of mRNA clinical subtypes [31] (Accession codes: E-TABM-158, E-TABM-276, E-TABM-66, GSE10797 , GSE11121 , GSE11965 , GSE12093 , GSE12306 , GSE12763 , GSE12917 , GSE13671 , GSE1456 , GSE1561 , GSE3494 , GSE4922 , GSE5460 , GSE5462 , GSE5764 , GSE5847 , GSE6532 , GSE6596 , GSE6883 , GSE7390 , GSE7904 , GSE8193 , GSE8977 , GSE9195 , GSE9574 ). Elevated Dicer expression and high cyclin D1 expression were significantly correlated with the luminal A subtype of breast cancer ( Fig. 5a , P <0.01, χ 2 -square test). Reduced Dicer expression and low level of cyclin D1a were significantly correlated with the basal-like breast cancer subtype ( Fig. 5b , P <0.05, χ 2 -square test). 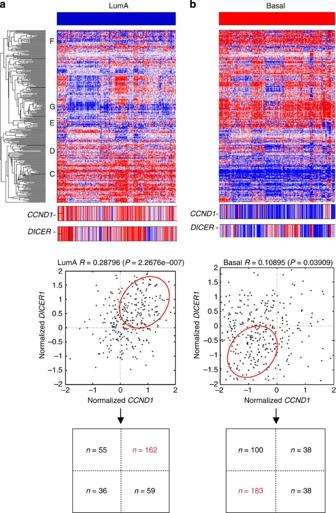Figure 5: A positive correlation analysis betweenDicerandcyclin D1aexpression in breast cancer patients. (a) Tree view display of gene expression from breast cancer patient samples for luminal A and basal genetic subtype. 2D-scatter plot for the elevatedDicerexpression and high expression ofcyclin D1ain luminal A breast cancer subtype (N=312). (b) 2D-scatter plot for the decreased Dicer expression and low expression ofcyclin D1ain basal breast cancer subtype (N=359). The number of breast cancer patient samples found in each of the four quadrants is indicated. Plots are labelled with Pearson’s correlation coefficient R and the correlationP-value. Figure 5: A positive correlation analysis between Dicer and cyclin D1a expression in breast cancer patients. ( a ) Tree view display of gene expression from breast cancer patient samples for luminal A and basal genetic subtype. 2D-scatter plot for the elevated Dicer expression and high expression of cyclin D1a in luminal A breast cancer subtype ( N =312). ( b ) 2D-scatter plot for the decreased Dicer expression and low expression of cyclin D1a in basal breast cancer subtype ( N =359). The number of breast cancer patient samples found in each of the four quadrants is indicated. Plots are labelled with Pearson’s correlation coefficient R and the correlation P -value. Full size image The current studies extend our prior findings that cyclin D1 regulates selected miRNAs at the transcriptional level in breast cancer [3] ( Fig. 6a ), by demonstrating that cyclin D1 induces Dicer expression and thereby governs pre-miRNA processing in human breast cancer ( Fig. 6b,c ). 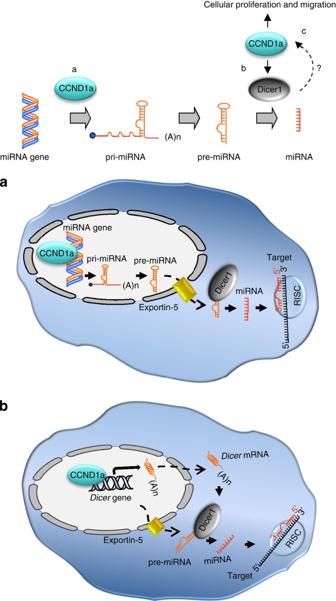Figure 6: Hypothetical Mechanisms for cyclin D1 regulation of miRNA abundance. Schematic representation of the hypothetical molecular mechanisms by which cyclin D1a induces miRNA expression (a) or processing (b) through inducing Dicer expression and promoting pre-miRNA to mature miRNA processing. In turn, Dicer may involve in the regulation of cell proliferation and migration by cyclin D1 (c). Figure 6: Hypothetical Mechanisms for cyclin D1 regulation of miRNA abundance. Schematic representation of the hypothetical molecular mechanisms by which cyclin D1a induces miRNA expression ( a ) or processing ( b ) through inducing Dicer expression and promoting pre-miRNA to mature miRNA processing. In turn, Dicer may involve in the regulation of cell proliferation and migration by cyclin D1 ( c ). Full size image The studies herein identify a novel mechanism governing Dicer abundance via transcriptional induction by cyclin D1. Transient or sustained expression of a cyclin D1 transgene targeted to the mammary gland in vivo was sufficient to induce Dicer1 mRNA and protein abundance. Herein, Dicer promoter activity was induced by a mutant of cyclin D1 incapable of recruiting an active kinase complex. Cyclin D1 regulates the expression of genes via kinase-dependent and kinase-independent mechanisms [21] . Phosphorylation and derepression of pRB, activates E2F-dependent signalling, whereas kinase-independent signalling involves binding of cyclin D1 through associated DNA sequence-specific binding transcription factors [3] , [18] , [19] . In the current studies cyclin D1 enrichment was identified at the Dicer regulatory region, with enrichment by ChIP at −728 to −655 region. This site does not contain an E2F site. The cyclin D1 binding region of the Dicer and miR-17/20 cluster promoter regulatory region were remarkably enriched for common TF-binding sites (SOX10, FOXD3, FOXA1, FOXA1, ZNF354C, ELK1, ELF5, ETS1, MafB, ZEB1) [3] . Previous studies demonstrated the cyclin D1-DNA bound form occupies the regulatory region of genes involved in DNA replication [19] and the miR-17/20 cluster promoter regulatory region [3] . The current studies extend prior studies by showing that cyclin D1 regulates the rate-limiting step in miRNA biogenesis ( Fig. 6a,b ). Herein cyclin D1 had a crucial role in Dicer-mediated functions including histone tri methylation, cellular proliferation and migration. Dicer −/− HCT116 cells (Dicer KO) or cyclin D1 siRNA treated HCT116, demonstrated reduced tri-m-H3K9 immunofluorescence as shown in Dicer −/− ES cells [25] , [26] . Cyclin D1 siRNA further reduced tri-m-H3K9, suggesting an additional Dicer-independent function for cyclin D1. This finding is consistent with previous publications in which cyclin D1 recruited the H3K9 histone methyltransferase Suv39 together with HP1 to chromatin in chromatin immune precipitation assays. Although cyclin D1 KD or cyclin D1 knock out, resulted in a partial reduction in Dicer abundance and would not therefore be expected to generate a geno- or phenocopy of Dicer deletion, the ability of cyclin D1 to induce cellular proliferation and cellular migration, was co-dependent upon Dicer, as cyclin D1 KD failed to reduce cellular proliferation or cellular migration in Dicer −/− HCT116 cells. What might be the biological function for cyclin D1-mediated induction of miRNA biogenesis via induction of Dicer abundance? Dicer expression is regulated by multiple signalling cascades. Although Dicer is ubiquitously expressed, regulation of its expression may control miRNA biogenesis in specific cellular contexts. Control of Dicer expression by TRBP, MITF [14] , PACT (double-stranded RNA dependent kinase (PKR) activator), KH type splicing regulatory protein (KSRP), and herein cyclin D1, may contribute to controlling miRNA biogenesis in local microenvironments. As cyclin D1 is a labile growth factor and oncogene-inducible protein, the relative abundance of cyclin D1 may transduce oncogenic and growth factor signalling to control miRNA biogenesis in these local microenvironments. Dicer expression is altered in a tumour type specific manner [32] , and herein was increased in luminal A breast cancer correlating with increased cyclin D1. As Dicer is essential for miRNA processing, the reduction in Dicer expression with reduced cyclin D1 levels in basal-like breast cancer may alter processing of pre-miRNA. Regulatory feedback loops between oncogenes and miRNAs control cell-cycle progression. In some cases miRNAs cooperate with transcription factors to regulate target gene expression [33] , [34] . The cyclin D1 a isoform’s 3′ UTR contains miRNA binding sites responsible for attenuation of cyclin D1 a abundance by multiple miRNAs including miR-17 and miR-20 (ref. 3 ). The expression of cell-cycle regulator genes including CDK s, myc , E2F and cyclin D1, are also regulated by miRNA. Collectively the current studies extend the repertoire of functions for the cyclin D1 gene from the previously described regulation of the coding genome products to coordinating biogenesis of the non-coding genome products. Transgenic mice Cyclin D1 − / − mice were maintained in our lab on a mixed C57B1/6 × 129/SvJ background. MMTV- Cyclin D1 transgenic mice were made by Dr Emmett V. Schmidt’s lab. The tetracycline inducible mammary epithelial cell-targeted cyclin D1a transgenic mice were established on FVB strain in our lab. MMTV-rtTA transgenic mice were made by Dr Lewis Chodosh’s lab. Eight to ten-weeks-old female mice was used for in vivo experiments. All mouse experiments were done in accordance with the guidelines for the care and use of laboratory animals at Thomas Jefferson University. Cell culture The cyclin D1 +/+ and cyclin D1 − / − MEFs were derived from WT and cyclin D1 knockout mice [35] . Dicer − / − HCT116 cells were originally from Dr Bert Vogelstein at Johns Hopkins University. MCF-7 cells were originally from ATCC, and maintained in our lab. All cells were cultured in DMEM containing penicillin and streptomycin (100 mg of each/l) and supplemented with 10% fetal bovine serum. Vectors The Dicer luciferase reporter [14] , Dicer expression vector [36] and cyclin D1 expression vectors [37] were obtained from labs as referenced. Basic-pGL3 luciferase reporter vector was from Promega. Human cyclin D1a, Cyclin D1b and cyclin D1 KE complementary DNAs (cDNAs) were cloned into the mouse stem cell virus-internal ribosome entry site-green fluorescent protein retrovirus vector at the EcoR I site. The ecotropic packaging vector, pSV- ψ – E-MLV which provides ecotropic packaging helper function, was used with retrovirus to infect cells. SiRNA transfection All siRNAs were from Qiagen. Target sequence for cyclin D1 siRNA was AACAAGCTCAAGTGGAACCTG. The target sequence for negative-control siRNA was AATTCTCCGAACGTGTCACGT; Lipofectamine RNAiMax (Invitrogen) was used to transfect siRNA following the manufacturer’s instructions. Gene reporter assays For cellular transfection with reporter DNA, actively growing cells were seeded on 12-well plates at a density of 1 × 10 5 cells per well. The next day, cells were co-transfected using lipofectamine 2000 (Invitrogen) with 0.5 μg of pGL3 and 0.1 μg of CMV/ß-galactosidase plasmid. Twenty-four hours after transfection, luciferase activities were measured by AutoLumat and normalized with ß-galactosidase. miRNA northern blot analysis Briefly, total RNA (10–20 μg per lane) was loaded on a 15% denaturing polyacrylamide gel and electophoresed at 200 V until the bromophenol blue approached the bottom. The RNA was transferred from the gel to Hybond-N+ membrane using a semi-dry transfer apparatus. DNA oligonucleotide probes (20–23 nt) were 5′ end labelled with [γ- 32 P]-ATP and hybridization was carried out using Rapid-Hyb buffer following the manufacturer’s instructions (Amersham, Piscataway, NJ). All DNA probes were synthesized by Integrated DNA Technologies. The probe sequences for miRNA northern analysis were as follows: miR-16: 5′-CGCCAATATTTACGTGCTGCTA-3′; let-7a: 5′-AACTATACAACCTACTACCTCA-3′; miR-17-5p: 5′-ACTACCTGCACTGTAAGCACTTTG-3′; miR-20a: 5′-CTACCTGCACTATAAAGCACTTTA-3′. Cell proliferation assay 4 × 10 3 cells per well were seeded into 96-well plate. At the indicated time points, MTT was used to stain cells for measuring cell proliferation. Wound-healing assay Cells were counted and plated in equal numbers in 12-well tissue culture plates to achieve 95% confluence. Thereafter, a vertical wound was created using a 0.1 μl pipette tip. The wounded wells were cultures in serum-reduced medium (0.5% fetal bovine serum). Images were captured at designated times to assess wound closure. Quantitative reverse-transcription PCR Total RNA was extracted with Trizol reagent (Life Technologies). For mRNA quantitative reverse-transcription PCR, the synthesized cDNA was reverse-transcribed with SuperScript II (Life Technologies) using random primer. For miRNA quantitative reverse-transcription PCR, first strand cDNA of miRNAs was prepared using the miRCURY LNA TM Universal cDNA Synthesis Kit (Product no: 203300) from Exiqon following the manufacturer’s instruction. Primer sets for real-time PCR of miR-16, miR-17, miR-20a, let-7a and 5S rRNA were purchased from Exiqon. The SYBR Green Master Mix was ABI product (Life Technologies). The ABI 7900 HT Sequence Detection System (Life Technologies) was used for quantitative real-time PCR assay. Primer sequences: Dicer, F: 5′ TGTGATCCAGAGGAATTGGA 3′, R: 5′ ACGGTCCACAGTCTACCACA 3′; CCND1, F: 5′ CAGAGGCGGAGGAGAACAAA 3′, R: 5′ ATGGAGGGCGGATTGGAA 3′; Exportin 5, F: 5′ GAAGATGAGGCTGCAGATGA 3′, R: 5′ CCCTTCTTTGAAACACAGCA 3′; ß-actin, F: 5′ TGACGGCCAGGTCATCACCATT 3′, R: 5′CTTGATCTTCATTGTGCTGG 3′. Analysis of transcript co-expression within public microarray Gene expression profiles were median-centered, scaled to unitary standard deviation and 2D-scatter plots were produced for Dicer versus cyclin D1 transcript expression in the luminal A subtype of breast cancer. The number of samples bound in each of the four quadrants around x =0 and y =0 was used to build a contingency table. The observed number of samples in each the four quadrants was assessed for significance by comparing against the expected distribution – the total number of samples in each quadrant, using a χ 2 -square test. Western blot analysis and immunohistochemical staining Whole-cell lysates (50 μg) were separated by 8–10% SDS–PAGE, and the proteins were transferred to nitrocellulose membrane using a semi-dry transfer apparatus (Bio-Rad). After being blocked in 5% milk (w/v) at room temperature for 1 h, the membranes were incubated at 4 °C overnight with primary antibodies. Following 1XPBST washing for three times (10 min per time), the membranes were incubated with secondary antibodies at room temperature for 1 h followed by same washing procedure and ECL (enhanced chemiluminescence) staining. The original blots for all western blots are shown in Supplementary Figs S6–S13 . The following antibodies were used for western blotting: anti-cyclin D1 (Ab3) from Neomarker (1:2,000); anti- Dicer (sc-136979,1:1,000), anti-β-actin (sc-47778, 1:3,000) and anti-β-tubulin (sc-9104, 1:2,000) were from Santa Cruz Biotechnology; anti-DGCR8 (no. 10996, 1:1,000) from Proteintech; anti-Argonaute 2 (C34C6, 1:1,000) from Cell Signaling; anti-Drosha (A301886, 1:1000) from Bethyl; and anti-M2 Flag from Sigma (1:2,000). Anti-Histone H3 (tri methyl K9) from Abcam was used in western blot (1:2,500) and in immunohistochemistry (1:100), with 4,6-diamidino-2-phenylindole co-staining. ChIP assay ChIP DNA was prepared using ChIP assay kit (Upstate Chemicon) following the manufacturer’s instruction. Briefly, three 10-cm plates of MCF-7 cells transduced with retroviral vector encoding cyclin D1 or control were fixed for 10 min with 37% paraformaldehyde (final concentration 1%). Unreacted formaldehyde was quenched with glycine. The cells were washed twice with ice-cold PBS and the pellets harvested in 3 ml of PBS with protease inhibitor cocktail. DNA fragmentation was achieved by sonicating for 35 cycles of 20 s each at maximum speed using OMNI-Ruptor 4000 (OMNI International, Inc). Immuno-precipitation (IP) was performed with 10 μg of anti-Cyclin D1 (SC-20044, Santa Cruz) and equivalent amount of mouse IgG as negative control. Precipitated DNA was analysed by quantitative real-time PCR using human Dicer promoter-specific primers: P1, F: 5′-AAGAAACACGGTTGCAGTTG-3′, R: 5′-TGGCTGGCTTAAAGAACATCT-3′; P2, F: 5′-CTGGAGACAGAGTGAGACTCC-3′, R: 5′-TGAGGTAGGTGCTGAAACTGC-3′; P3, F: 5′-AACAGGAAGCAGGCTGGGTA-3′, R: 5′-CGATTTCTGACCTTGTCATC-3′; P4, F: 5′-CTTATTTAACGCCCACCGAT-3′, R: 5′-CCTGGCAGACCCATGTATTT-3′; P5, F: 5′-ACAAAGGGCATATCTTGGCT-3′, R: 5′-TGTCCCTCACACCTGTCCTA-3′; P6, F: 5′-AAACAAACCAGCAAGTGGAG-3′, R: 5′-TGGCTACACAGTCATTTATTGAG-3′. Statistical analysis Data are presented as mean±s.e.m. The standard two-tailed Student’s t -test was used for analysis and P <0.05 was considered significant. How to cite this article: Yu, Z. et al. Cyclin D1 induction of Dicer governs microRNA processing and expression in breast cancer. Nat. Commun. 4:2812 doi: 10.1038/ncomms3812 (2013).